Molecular protein adaptor with genetically encoded interaction sites guiding the hierarchical assembly of plasmonically active nanoparticle architectures The control over the defined assembly of nano-objects with nm-precision is important to create systems and materials with enhanced properties, for example, metamaterials. In nature, the precise assembly of inorganic nano-objects with unique features, for example, magnetosomes, is accomplished by efficient and reliable recognition schemes involving protein effectors. Here we present a molecular approach using protein-based ‘adaptors/connectors’ with genetically encoded interaction sites to guide the assembly and functionality of different plasmonically active gold nanoparticle architectures (AuNP). The interaction of the defined geometricaly shaped protein adaptors with the AuNP induces the self-assembly of nanoarchitectures ranging from AuNP encapsulation to one-dimensional chain-like structures, complex networks and stars. Synthetic biology and bionanotechnology are applied to co-translationally encode unnatural amino acids as additional site-specific modification sites to generate functionalized biohybrid nanoarchitectures. This protein adaptor-based nano-object assembly approach might be expanded to other inorganic nano-objects creating biohybrid materials with unique electronic, photonic, plasmonic and magnetic properties. The precise assembly of molecular structures and nano-objects in space bridging the scale from a few to several hundred nm is one of the key challenges in nanotechnology. Especially defined architectures of metallic nano-objects allow to create materials with new physical and chemical properties and effects. Therefore, great efforts have been devoted towards the spatial organization of metallic nanoparticles (NP) because of their potential applications in optics [1] , electronics [2] , magnetics [3] , biosensing [4] and energy conversion [5] . The ability to understand and control position, orientation and geometry of nano-objects such as NPs assembled with nanoscale precision is crucial to tune unique properties such as subwavelength optical guiding [6] or catalytics [7] . Current technologies and methods used to create nanoarchitectures include top down approaches such as e-beam lithography enabling structures down to 2-nm resolution [8] , pattern transfer processes such as etching [9] and bottom up approaches using dip-pen nanolithography (down to 30 nm resolution) [10] , hard-tip soft-spring lithography (with sub-50 nm resolution) [11] , self-assembly of nano-objects [12] and molecular e-beam epitaxy [9] . So far, it has been shown that one-dimensional (1D) gold NP (AuNP) structures can be achieved by template-free assemblies such as chemical bonding [13] , [14] , hydrogen bonding [15] , electrostatic forces and van der Waals forces. Such assemblies have been induced by small organic molecules, for example, mercapthoethanol [16] and destabilizing agents as salt [17] or ethanol [18] . Recently, bioinspired approaches utilizing the advantages of biological constituents for template-based assembly of nanoarchitectures have gained considerable attention [19] , [20] . In this context, a template can be defined as a geometrical object significantly larger than the NP to be deposited. The most widely used biological template for directed AuNP assemblies is DNA [21] , [22] , but also peptide fibrils [23] or protein fibres [2] were deployed as templates, for example, amyloid fibres for the construction of conducting nanowires [2] . Another prominent example for proteinaceous assemblies is the patterning or encapsulation of metal NPs by virus capsids [24] , [25] , [26] . The great advantage of protein-based assemblies is the ability to store and tune information about precise structure, composition and interaction potential on the genetic level. Here we focus on another high-resolution bottom up approach, the protein adaptor-based nano-object assembly (PABNOA), which leads to protein-guided self-assembly of NPs. The adaptor-based strategy fundamentally differs from known template-based nano-object assembly strategies. It directly connects nano-objects via adaptor complexes of roughly the same size as the nano-object, which is in contrast to template-based strategies where the dimension of the template is much larger than the nano-objects to be assembled. The bioinspired translation of genetic information into biomimetic nanostructures enables to guide the self-assembly of genetically encoded protein-based nanoscale biohybrid materials. Existing methods involve proteins to assemble nanostructures of defined shape usually by using the protein as a template to assemble NPs, for example, around spherical virus capsids or along protein fibre scaffolds. One of the very few template-free protein-based NP organization schemes is reported for streptavidin/biotin [27] -induced NP assembly. In contrast, we focus on developing a geometrically defined protein-building block to connect NP specifically. In this article we introduce the idea of an active NP-connecting process utilizing proteins with defined geometrical shape as adaptors, allowing to assemble and organize nano-objects in space. This biotechnological approach is realized using toroidal, donut-shaped proteins (Hcp1) as molecular adaptors with defined geometric shape and defined localization and orientation of functional groups including unnatural amino acids for site-selective modification. This PABNOA shows template-free self-assembly of different plasmonically active AuNP nanoarchitectures. We characterize the mechanism, plasmonic coupling, chain length, protein-NP surface coverage and site-specific organic dye functionalization via transmission electron microscopy (TEM), fluorescence microscopy and UV–vis spectrometry. Therefore, a newly cloned library of toroidal Hcp1 mutants is generated and screened regarding their potential to guide self-assembly processes. Toroidal protein adaptor-building blocks for NP organization Creating nanoarchitectures via structurally and functionally defined protein structures connecting and ordering nano-objects such as NPs requires the design and (bio)synthesis of functional proteins. In this work, we use the toroidal Hcp1 pore protein from Pseudomonas aeruginosa and different-sized AuNPs as major building blocks for various self-assembled nanoarchitectures. AuNPs ranging from 3 to 40 nm in diameter capped with different ligands were purchased or synthesized [28] . 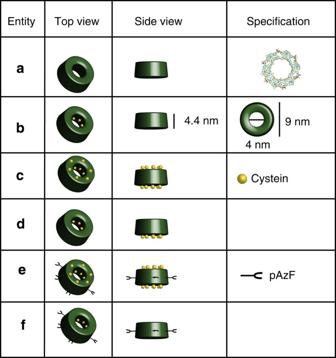Figure 1: Newly designed functional library of Hcp1 mutants. (a) Hcp1 wt and Hcp1wt crystal structure (pdb entry 1y12)29. (b) Hcp1_Q54C bearing a cysteine at the inner cavity at the solvent-accessible position 54. (c) Hcp1_Q54C_G91C_N159C (Hcp1_cys3)-bearing thiols at upper and lower rim and inside the cavity. (d) Hcp1_Q54C_N159C with a thiol at the lower and inner rim only. (e) Hcp1_cys3_D11pAzF bearing three additional thiols per monomer and the genetically encoded unnatural amino-acid pAzF introduced in the middle of the outer ring surface of the protein donut. (f) Hcp1_Q54C_D11pAzF containing a cysteine inside the cavity and the genetically encoded unnatural amino acid pAzF introduced in the middle of the outer ring surface of the protein donut. For all experiments, 5 and 10 nm AuNPs with a mixed tannic-citric acid ligand and 40 nm AuNPs with citric acid ligand were used, if not stated otherwise (for details see Supplementary Table 1 ). Hcp1 was expressed in large scale in E. coli and purified via a Ni-NTA column with a yield of ~0.03–0.16 mg ml −1 cell culture (dependent on the mutant). Hcp1 is a torus ring-shaped homo-hexameric pore protein of 112 kDa with an outer diameter of 9.0 nm, an inner diameter of 4.0 nm and a height of 4.4 nm. Hence, it is suitable as toroidal/donut-shaped protein adapter for 3D NP assembly ( Fig. 1a ) [29] . Owing to its defined geometrical shape, it has been used and characterized as nanotechnological building block for protein fibres [30] , [31] and the assembly of quantum dot biohybrid structures by our group [32] . Figure 1: Newly designed functional library of Hcp1 mutants. ( a ) Hcp1 wt and Hcp1wt crystal structure (pdb entry 1y12) [29] . ( b ) Hcp1_Q54C bearing a cysteine at the inner cavity at the solvent-accessible position 54. ( c ) Hcp1_Q54C_G91C_N159C (Hcp1_cys3)-bearing thiols at upper and lower rim and inside the cavity. ( d ) Hcp1_Q54C_N159C with a thiol at the lower and inner rim only. ( e ) Hcp1_cys3_D11pAzF bearing three additional thiols per monomer and the genetically encoded unnatural amino-acid pAzF introduced in the middle of the outer ring surface of the protein donut. ( f ) Hcp1_Q54C_D11pAzF containing a cysteine inside the cavity and the genetically encoded unnatural amino acid pAzF introduced in the middle of the outer ring surface of the protein donut. Full size image In order to study, control and fine-tune the self-assembly potential of Hcp1 and AuNPs, geometrically controlled interaction sites were introduced into each monomer of the hexameric protein structure. Taking advantage of the strong gold–thiol interaction of ~45 kcal mol −1 , cysteins have been introduced into the 3D protein structure as NP-anchor points. At strategic positions, for example, at the plane of the ‘ring face’ of the protein-‘donut’, these ‘guiding points’ allow for the directed self-assembly of AuNP and Hcp1 ‘donuts’. Subsequently, a functional library of Hcp1 mutants was designed ( Fig. 1 ) containing: (a) Hcp1 wild type (wt) bearing only one cysteine per monomer, which is not solvent-accessible, (b) Hcp1_Q54C where at the inner cavity glutamic acid (Q) was exchanged for cysteine (C) at the solvent-accessible position 54, (c) Hcp1_Q54C_G91C_N159C (Hcp1_cys3) bearing thiols at the lower and upper rim and inside the cavity of the protein donut and (d) Hcp1_Q54C_N159C with a thiol at the lower rim only. Expanding the functionality of the protein library ( Fig. 1e,f ) a genetically encoded unnatural amino acid (UAA) was introduced at the outer surface of the torus protein ring via the amber suppression method [33] . By replacing aspartic acid (D) at position 11 with p -azidophenylalanine (D11pAzF), a new bioorthogonal interaction side allows for site-specific conjugation, for example, with fluorescent entities, interacting with the plasmonic field of the AuNPs. The successful incorporation of pAzF was proven using LC-MS/MS and SDS–PAGE ( Supplementary Fig. 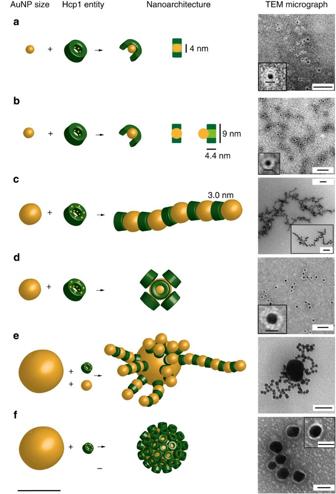Figure 2: Self-assembled nanoarchitectures induced by different Hcp1 mutants and AuNP sizes. (a) Four-nanometre AuNPs incorporated and stabilized by Hcp1_Q54C. (b) Five-nanometre AuNPs partly incorporated and stabilized by Hcp1_Q54C. (c) Hcp1_cys3 addition to a solution of 10 nm AuNPs leads to 1D network formation. (d) Incubation of an excess of Hcp1_cys3 with 10 nm AuNPs (capped with citrate ligand only) leads to a full surface coverage of 10 nm AuNPs. (e) Hcp1_cys3 initialized chain growth of 10 nm AuNPs and subsequent addition of 40 nm AuNPs leads to the formation of hedgehog-like structures containing 40 nm AuNPs and branching chains of 10 nm AuNPs. (f) Incubation of an excess of Hcp1_cys3 with 40 nm AuNPs (capped with citric acid ligand only) leads to a full surface coverage of 40 nm AuNPs. Thiols on the rim sides are not shown for better visibility. Imaging of all structures shown inFig. 2(except ine) involved negative staining with uranyl formate. Scale bars of all micrographs, 50 nm except micrograph insertsa,b,dcorrespond to 10 nm. Scale bar scheme, 40 nm. 1 , Supplementary Note 1 , Supplementary Table 2 ). The bio-orthogonally reactive azide moiety (D11pAzF), thiols inside the cavity (Hcp1_Q54C_D11pAzF, Fig. 1f ) as well as at the upper and the lower sites of the rim (Hcp1_cys3_D11pAzF, Fig. 1e ) in one hexameric building block, generate new multivalent protein-based adapter molecules. The application of these complex adaptor proteins will be discussed in detail in the last section of this paper. Self-assembled nanoarchitectures guided by protein adaptors The Hcp1 mutants introduced in Fig. 1 were applied to guide the assembly of various AuNP-Hcp1 nanostructures. First, the addition of Hcp1_Q54C to a solution of 3- to 5-nm-sized AuNPs leads to a direct incorporation of the AuNPs into the protein cavity. TEM micrographs in Fig. 2a,b indicate the negatively stained (bright) protein ring around the 3- to 5-nm-sized dark AuNPs in appropriate dimensions (~2.5 nm). In total, six genetically engineered thiols ( Fig. 1b ) of the hexameric ring attach the 3-nm AuNP entirely inside the cavity ( Fig. 2a ). For the structural arrangement of the 5-nm AuNP, two conformations are possible ( Fig. 2b ). In assumption of a flexible protein ring, the 5-nm AuNP might be incorporated entirely. In contrast, a rigid structure would only allow for an AuNP-penetration of ~1 nm (for details see Supplementary Note 2 ). Even though a strong central binding of the 5-nm AuNP inside the cavity is evident (TEM image of Fig. 2b ), the penetration distance of the particle cannot be entirely resolved via TEM. Figure 2: Self-assembled nanoarchitectures induced by different Hcp1 mutants and AuNP sizes. ( a ) Four-nanometre AuNPs incorporated and stabilized by Hcp1_Q54C. ( b ) Five-nanometre AuNPs partly incorporated and stabilized by Hcp1_Q54C. ( c ) Hcp1_cys3 addition to a solution of 10 nm AuNPs leads to 1D network formation. ( d ) Incubation of an excess of Hcp1_cys3 with 10 nm AuNPs (capped with citrate ligand only) leads to a full surface coverage of 10 nm AuNPs. ( e ) Hcp1_cys3 initialized chain growth of 10 nm AuNPs and subsequent addition of 40 nm AuNPs leads to the formation of hedgehog-like structures containing 40 nm AuNPs and branching chains of 10 nm AuNPs. ( f ) Incubation of an excess of Hcp1_cys3 with 40 nm AuNPs (capped with citric acid ligand only) leads to a full surface coverage of 40 nm AuNPs. Thiols on the rim sides are not shown for better visibility. Imaging of all structures shown in Fig. 2 (except in e ) involved negative staining with uranyl formate. Scale bars of all micrographs, 50 nm except micrograph inserts a , b , d correspond to 10 nm. Scale bar scheme, 40 nm. Full size image Another major objective was to achieve not only incorporation of AuNPs into the toroidal protein cavity but also successful linear assembly of Hcp1–AuNP conjugates. Therefore, we decided to use the Hcp1_cys3 mutant ( Fig. 1c ) with gold-reactive upper and lower interaction sites in combination with 10-nm AuNPs, which are in the range of the protein diameter (9.5 nm). Accordingly, the interaction between Hcp1_cys3 ( Fig. 2c ) and 10-nm AuNPs leads to 1D chains and network formation, clearly visible in the TEM images ( Figs 2c , 3 and 4 ). The self-assembly potential of other Hcp1 mutants as negative controls ( Fig. 1 ) was tested as well. Neither Hcp1 wild type nor Hcp1_Q54C or Hcp1_Q54C_N159C induce NP assembly ( Supplementary Fig. 2 ). These Hcp1 mutants evidenced AuNP binding, which can be deduced from small surface plasmon resonance (SPR) shifts, recorded via UV–vis spectrometry. However, no AuNP assembly is observed on the respective TEM micrographs ( Supplementary Fig. 2 ). Therefore, thiols on both rim sides of Hcp1_cys3 ( Fig. 1c ) are the essential driving force for the chain formation discussed in detail below. Additional cryo-TEM micrographs ( Supplementary Fig. 3 ) reveal the same AuNP chain morphology as samples imaged via conventional TEM. Therefore, drying and imaging artefacts through sample preparation can be excluded. 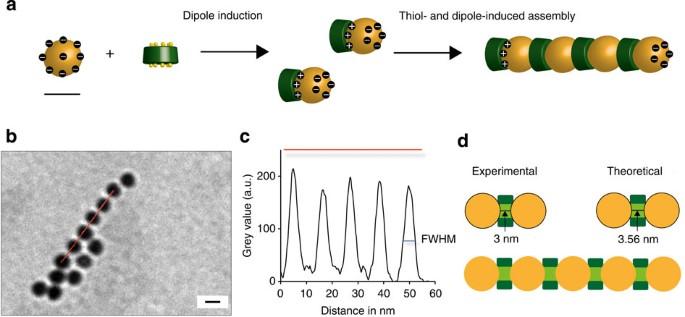Figure 3: Mechanism of the protein adaptor–AuNP assembly. (a) Illustration of the proposed two-step assembly mechanism: first, Hcp1_cys3 binding through thiol-anchoring points induces anisotropic ligand distributions, which results in dipole formation. Second, multiple dipole–dipole interactions and Hcp1_cys3 binding leads to stable AuNP chains. (b,c) The plot profile of the interparticle distances of assembled AuNPs on a TEM micrograph is shown. (d) The experimental measurement of the full-width half maximum (FWHM) ofn=73 AuNP distances yielded a mean value of 3.0±0.5 nm. The scheme illustrates the theoretical distance value of 3.56 nm for a perfect spherical ball and a rigid ring. Scale bar ina,b, 10 nm. Figure 3: Mechanism of the protein adaptor–AuNP assembly. ( a ) Illustration of the proposed two-step assembly mechanism: first, Hcp1_cys3 binding through thiol-anchoring points induces anisotropic ligand distributions, which results in dipole formation. Second, multiple dipole–dipole interactions and Hcp1_cys3 binding leads to stable AuNP chains. ( b , c ) The plot profile of the interparticle distances of assembled AuNPs on a TEM micrograph is shown. ( d ) The experimental measurement of the full-width half maximum (FWHM) of n =73 AuNP distances yielded a mean value of 3.0±0.5 nm. The scheme illustrates the theoretical distance value of 3.56 nm for a perfect spherical ball and a rigid ring. Scale bar in a , b , 10 nm. 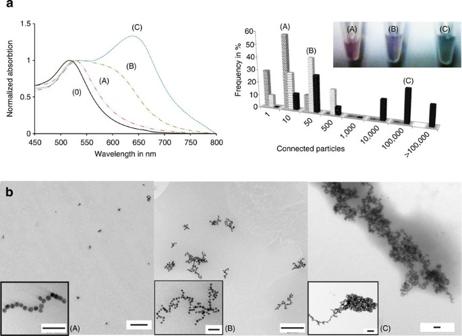Figure 4: AuNP chain assembly guided by the stoichiometry of Hcp1/AuNP and the addition/mixing protocol. (a) On the left side, depicted are UV–vis spectra of assembled structures under different assembly conditions. The conditions are labelled with (A) for fast addition and mixing of 40 eq Hcp1_cys3, (B) slow addition and mixing of 5 eq Hcp1_cys3, (C) punctual addition (no mixing) of 2 eq Hcp1_cys3 and (O) for pure 10 nm AuNP in solution without protein. The graph on the right side illustrates the particle length distribution: eight length classes with a five decade span were defined and the frequency distribution of the number of connected particles for each assembly condition A, B and C is shown. The images depict the macroscopically visible colour change from red to pale pink depending on the assembly condition. (b) From left to right, representative TEM micrographs illustrate the different chain length for the assembly condition A, B and C. Scale bars inb, 200 nm and for inserts 50 nm except for right image insert, 200 nm. Full size image Figure 4: AuNP chain assembly guided by the stoichiometry of Hcp1/AuNP and the addition/mixing protocol. ( a ) On the left side, depicted are UV–vis spectra of assembled structures under different assembly conditions. The conditions are labelled with (A) for fast addition and mixing of 40 eq Hcp1_cys3, (B) slow addition and mixing of 5 eq Hcp1_cys3, (C) punctual addition (no mixing) of 2 eq Hcp1_cys3 and (O) for pure 10 nm AuNP in solution without protein. The graph on the right side illustrates the particle length distribution: eight length classes with a five decade span were defined and the frequency distribution of the number of connected particles for each assembly condition A, B and C is shown. The images depict the macroscopically visible colour change from red to pale pink depending on the assembly condition. ( b ) From left to right, representative TEM micrographs illustrate the different chain length for the assembly condition A, B and C. Scale bars in b , 200 nm and for inserts 50 nm except for right image insert, 200 nm. Full size image The structural diversity of the NP architectures was further expanded by assembling different NP sizes ( Fig. 2e ). When chain growth of 10 nm AuNPs is initialized by addition of Hcp1_cys3 and subsequently 40 nm AuNPs are added, hedgehog-like structures of 40 nm AuNPs with chains of 10 nm AuNPs can be grown and were analysed via TEM ( Fig. 2e ) and UV–vis ( Supplementary Fig. 4a–c ). Control samples containing 40- and 10-nm AuNPs but lacking Hcp1_cys3 did not show chain formation but rather unspecific agglomerates ( Supplementary Fig. 4d,e ). A complete functionalization of 10- and 40-nm AuNPs with a distinct number of Hcp1_cys3 molecules could be monitored with TEM images and with UV–vis spectrometry (described in Fig. 5 ). On negative staining, TEM images clearly reveal the presence of the protein-donut corona in corresponding dimensions constituting Hcp1_cys3 ( Fig. 2d,f ). These protein-shelled AuNPs are long-term stable (tested for 2 months), even after addition of 250 mM NaCl, and might be used as platform for the selective modification with functional molecules as described in Fig. 6 . 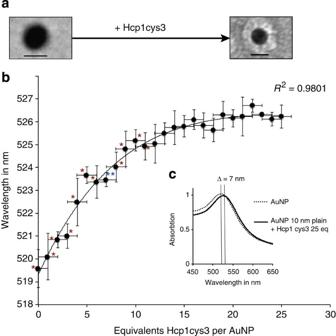Figure 5: Monitoring the Hcp1_cys3 surface coverage of 10 nm AuNPs. (a) TEM images (negatively stained) of plain 10 nm AuNP and fully Hcp1_cys3-covered AuNPs. (b) Wavelengths of the SPR peaks of a 10 nm AuNP solution as function of the number of equivalents (1–25 eq) of Hcp1_cys3 hexamers added to the solution. The fitted regression curve and its asymptotic progression atx=25 eq correspond to a full surface coverage of the AuNP. Error bars indicate the s.d. of the mean and the statistical significance (withP<0.05) is indicated with * for those values (λ=1–11), which are significantly different from the asymptotic maximum (25 eq, 526.4 nm). The first value being significantly (P<0.05) different from (λ=11) is indicated with** (λ=7).t-test and error analysis (Supplementary Note 6) indicate that ~9±3.04 eq Hcp1_cys3 are needed to cover the whole surface of a 10-nm AuNP. (c) UV–vis extinction spectrum of a solution with plain 10 nm AuNPs and the addition of 25 eq Hcp1_cys3 leads to an SPR shift of ~7 nm. Scale bar ina, 10 nm. Figure 5: Monitoring the Hcp1_cys3 surface coverage of 10 nm AuNPs. ( a ) TEM images (negatively stained) of plain 10 nm AuNP and fully Hcp1_cys3-covered AuNPs. ( b ) Wavelengths of the SPR peaks of a 10 nm AuNP solution as function of the number of equivalents (1–25 eq) of Hcp1_cys3 hexamers added to the solution. The fitted regression curve and its asymptotic progression at x =25 eq correspond to a full surface coverage of the AuNP. Error bars indicate the s.d. of the mean and the statistical significance (with P <0.05) is indicated with * for those values ( λ =1–11), which are significantly different from the asymptotic maximum (25 eq, 526.4 nm). The first value being significantly ( P <0.05) different from ( λ =11) is indicated with** ( λ =7). t -test and error analysis ( Supplementary Note 6 ) indicate that ~9±3.04 eq Hcp1_cys3 are needed to cover the whole surface of a 10-nm AuNP. ( c ) UV–vis extinction spectrum of a solution with plain 10 nm AuNPs and the addition of 25 eq Hcp1_cys3 leads to an SPR shift of ~7 nm. Scale bar in a , 10 nm. 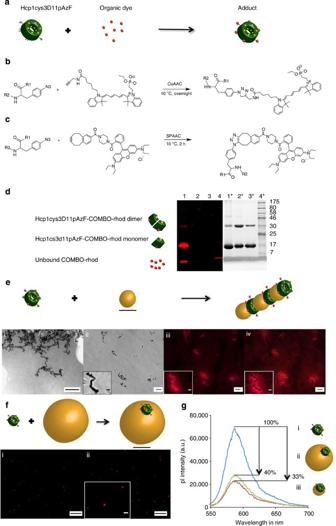Figure 6: The bioorthogonal modification of bifunctional Hcp1_cys3_D11pAzF. (a) Reaction between organic dye and unnatural amino acid pAzF, which was co-translationally incorporated into Hcp1. (b) CuAAC: copper-catalysed azide-alkyne-cycloaddition between Hcp1_cys3_D11pAzF and the alkyne dye 642 in the presence CuSO4, THPTA ligand and sodium ascorbat at 10 °C overnight. (c) SPAAC: strain-promoted cycloaddition of azide and cyclooctyne between Hcp1_cys3_D11pAzF and COMBO-rhod at 10 °C for 2 h. (d) SDS–PAGE of Hcp1_cys3_D11pAzF reacted with COMBO-rhod after excitation of COMBO-rhod (left) and the same gel stained with Coomassie-Brilliant Blue (right). Lanes 1–4 show (1) Hcp1_cys3_D11pAzF-COMBO-rhod, (2) Control Hcp1_wt incubated with COMBO-rhod, (3) Hcp1_wt and (4) Proteinladder 7–175 kDa with one fluorescent protein at 7 kDa. Successful cycloaddition between COMBO-rhod and Hcp1_cys3_D11pAzF is confirmed by the red fluorescent bands in lane 1 showing the monomer and dimer of Hcp1 with the attached red dye (red arrow). (e) Illustration of Hcp1_cys3_D11pAzF-COMBO-rhod and 10-nm AuNP chain assembly. Formed architectures are imaged (i) via TEM by (ii) light microscopy and (iii) fluorescence microscopy. (iv) Superimposed images of (ii)+(iii) show strong quenching of the attached rhodamin dye due to dye–AuNP–SPR interaction. (f) Scheme of dye-labelled Hcp1_cys3_D11pAzF bound to individual 40-nm AuNPs (for better visibility only one of multiple attachments are shown). Fluorescence images of (i) Hcp1_cys3_D11pAzF-COMBO-rhod and (ii) Hcp1_cys3_D11pAzF—alkyne dye 642 bound to 40-nm AuNPs show single fluorescent spot with a strong blinking behaviour (seeSupplementary Movie 1). (g) Fluorescence spectroscopy measurements of (i) Hcp1_cys3_D11pazF-COMBO-rhod, (ii) Hcp1_cys3_D11pazF-COMBO-rhod bound to 40 nm AuNPs and (iii) Hcp1_cys3_D11pazF-COMBO-rhod bound to 10 nm AuNPs reveals 60 and 67% quenching, respectively. Scale bar in illustratione, 10 nm, micrograph (i) 100 nm, (ii–iv) 5 μm and inserts 1 μm. Scale bars in scheme (f), (i) and (ii), 10 μm, and insert (ii), 1 μm. Full size image Figure 6: The bioorthogonal modification of bifunctional Hcp1_cys3_D11pAzF. ( a ) Reaction between organic dye and unnatural amino acid pAzF, which was co-translationally incorporated into Hcp1. ( b ) CuAAC: copper-catalysed azide-alkyne-cycloaddition between Hcp1_cys3_D11pAzF and the alkyne dye 642 in the presence CuSO 4 , THPTA ligand and sodium ascorbat at 10 °C overnight. ( c ) SPAAC: strain-promoted cycloaddition of azide and cyclooctyne between Hcp1_cys3_D11pAzF and COMBO-rhod at 10 °C for 2 h. ( d ) SDS–PAGE of Hcp1_cys3_D11pAzF reacted with COMBO-rhod after excitation of COMBO-rhod (left) and the same gel stained with Coomassie-Brilliant Blue (right). Lanes 1–4 show (1) Hcp1_cys3_D11pAzF-COMBO-rhod, (2) Control Hcp1_wt incubated with COMBO-rhod, (3) Hcp1_wt and (4) Proteinladder 7–175 kDa with one fluorescent protein at 7 kDa. Successful cycloaddition between COMBO-rhod and Hcp1_cys3_D11pAzF is confirmed by the red fluorescent bands in lane 1 showing the monomer and dimer of Hcp1 with the attached red dye (red arrow). ( e ) Illustration of Hcp1_cys3_D11pAzF-COMBO-rhod and 10-nm AuNP chain assembly. Formed architectures are imaged (i) via TEM by (ii) light microscopy and (iii) fluorescence microscopy. (iv) Superimposed images of (ii)+(iii) show strong quenching of the attached rhodamin dye due to dye–AuNP–SPR interaction. ( f ) Scheme of dye-labelled Hcp1_cys3_D11pAzF bound to individual 40-nm AuNPs (for better visibility only one of multiple attachments are shown). Fluorescence images of (i) Hcp1_cys3_D11pAzF-COMBO-rhod and (ii) Hcp1_cys3_D11pAzF—alkyne dye 642 bound to 40-nm AuNPs show single fluorescent spot with a strong blinking behaviour (see Supplementary Movie 1 ). ( g ) Fluorescence spectroscopy measurements of (i) Hcp1_cys3_D11pazF-COMBO-rhod, (ii) Hcp1_cys3_D11pazF-COMBO-rhod bound to 40 nm AuNPs and (iii) Hcp1_cys3_D11pazF-COMBO-rhod bound to 10 nm AuNPs reveals 60 and 67% quenching, respectively. Scale bar in illustration e , 10 nm, micrograph (i) 100 nm, (ii–iv) 5 μm and inserts 1 μm. Scale bars in scheme ( f ), (i) and (ii), 10 μm, and insert (ii), 1 μm. Full size image Characteristics of protein adaptor AuNP assembly In order to investigate and evolve the mechanism and characteristics of the complex self-assembly process of Hcp1_cys3–10 nm and AuNP, assembled biohybrid structures were investigated in depth. As mentioned before, electrostatic interactions, van der Waals forces and the dipolar interaction potential of AuNPs play a crucial role for the assembly process of NPs [17] , [34] , [35] . Heterogeneities in surface charge and polarity are the main results of anisotropic ligand organizations, leading to dipole formation and finally resulting in anisotropic AuNP assemblies [34] . As reported by other groups [16] , [36] , a partial ligand exchange (for example, ß-mercaptoethanol against negatively charged citrate/citric acid) progressively reduces electrostatic repulsion and induces electric dipole formation. For our system, a similar mechanism is proposed, even though induced by a complex protein-aqueous ring structure ( Fig. 3a ). As Hcp1_cys3 is binding AuNPs on one rim side, a partial ligand exchange (preferably tannic acid) induces dipole formation and short-range anisotropic dipole attraction forces enabling the binding of the thiols of Hcp1_cys3 to a second adjacent AuNP, which ultimately leads to 1D chain growth. It is important to note that exclusively the triple mutant Hcp1_cys3 with thiols on both sides of the donut rim does induce the formation of NP architectures via the strong thiol–gold interaction. Even though Hcp1_cys3 binds the 10-nm AuNPs of different ligands (for example, citrate-stabilized and citrate-tannic acid-stabilized) as proven with TEM and UV–vis spectrometry ( Figs 2 and 4 ) only the 10-nm AuNPs with a mixed ligand composition of tannic acid and citrate [37] show self-assembly into chain- and network-like structures without the addition of organic solvent or salt. In contrast, 10-nm AuNPs with citrate ligand only show self-assembly and chain formation after lowering the dielectric constant of the solvent (for details see Supplementary Note 3 and Supplementary Fig. 5 ). Further elucidation of the proposed mechanism and the function of Hcp1_cys3 as protein adapter between adjacent AuNPs could be achieved with detailed TEM and UV–vis analyses of the formed AuNP chain assemblies. The AuNP-Hcp1_cys3 surface coverage, the change of the anisotropic behaviour (by varying the assembly conditions), the associated chain length and plasmonic coupling of the AuNP architectures has been investigated and is described below. On all related TEM images ( Figs 2c , 3b and 4c–e ) a clearly visible space between the aligned AuNPs is observed, demonstrating the function and presence of the protein adapter Hcp1_cys3 as geometric adaptor/connector between the individual 10-nm AuNPs. If compared with AuNP assemblies induced by small organic molecules or organic solvents no such defined spacing between NPs can be observed [16] , [38] . Assuming a rigid gold sphere with perfect spherical shape of r AuNP =5 nm with x =2 nm as the radius of the void inner cavity of the Hcp1_cys3 protein ring, a maximal penetration distance of the sphere into the protein ring is calculated to be 0.42 nm (for details see Supplementary Note 2 ). According to the crystal structure, Hcp1_cys3 is 4.4 nm in height; hence, the theoretical maximal interparticle distance can be predicted to be 3.56 nm ( Fig. 3d ). Experimentally, the maximal distance of 1D aligned interacting AuNPs, was measured to be 3.0 nm±0.5 nm ( Fig. 3b,c ). This value is in very good agreement with the calculated theoretical distance of 3.56 nm. The small difference between these values can be explained by the flexibility of the protein ring allowing for deeper penetration of the AuNPs, the geometrical shape and size of the AuNPs differing from the assumption for the calculation of perfectly symmetric 10-nm AuNPs, a deviation from the 180° AuNP assembly axis of the AuNP chain and experimental constraints like the drying process on the TEM grid. During the self-assembly of Hcp1_cys and 3–10 nm AuNPs, a distinct colour change of the AuNP solution from pale pink to pale blue can be observed by eye and monitored via UV–vis spectrometry ( Fig. 4a ). The localized surface plasmon of individual AuNPs of 10 nm can be visualized by the absorption band at ~520 nm ( Fig. 4a ). After the addition of Hcp1_cys3 to a 10-nm AuNP solution a strong second signal at ~600 nm evolves, which results from a strong longitudinal plasmonic coupling ( Fig. 4a ), similar to those reported elsewhere [36] . Hence, chain formation is associated with a strong contact-free plasmonic coupling of the 10 nm AuNPs through Hcp1_cys3 and ultimately leads to a plasmonically active NP network ( Fig. 4 ). Macroscopically, the assembly process can be tracked by the observation of a slowly developing colour change from the point of protein addition. TEM and UV–vis spectrometry indicate for a fast assembly process of different NP architectures. The shifted plasmon band is stable and chain-like assemblies are observed within 1 min after protein addition. Once the AuNPs are functionalized with Hcp1_cys3 these assemblies are stable for weeks at room temperature without any agglomeration or precipitation. In contrast, Hcp1_wt ( Supplementary Fig. 2a (iv)) adsorbs on AuNPs unspecifically, as proven by the SPR shift and agglomerates are visible within 2 h after addition. The knowledge about the anisotropic AuNP assembly process has been used to guide the chain and network formation and the plasmonic properties of the formed architectures. As mentioned above, AuNP chain assembly is driven by Hcp1_cys3-induced dipole attraction forces. Hence, by changing the number of anisotropic AuNPs the resulting assembled structures can be varied. Therefore, the following variables seem to be important: the ligand of the NPs, the stoichiometry of Hcp1_cys3 per AuNP and the mixing scheme, the solvent and the ion concentration in the solvent (the dielectric constant of the solvent and the ion concentration alter the Debye screening length) and the ratio of the volumes of the components to be mixed. The influence of these variables on the NP assembly and their plasmonic properties have been monitored macroscopically via UV–vis spectrometry and TEM. A distinct correlation between the intensity of the red-shifted SPR band and the extent of chain and network is confirmed via TEM ( Fig. 4 ) and has also been shown by other groups [16] , [36] , [39] . High protein ratios per NP (for example, 40 eq (equivalent) Hcp1_cys3) and fast mixing after addition leads to a small intensity of the red-shifted longitudinal SPR band, a red pale solution and short NP chains (no loops or networks; Fig. 4 assembly condition A). As the equivalents of Hcp1_cys3/NP are decreased, for example, to 5 eq and mixing after addition is delayed, the intensity of the red-shifted longitudinal band does increase ( Fig. 4 assembly condition B). This is also visible by a colour change from pale red to pale red-pink. The observed AuNP chain length, AuNP loops and branched chains on the TEM micrographs are extended ( Fig. 4 assembly condition B). Finally, a pronounced intensity of the red-shifted longitudinal SPR band corresponds to a pale pink solution and an extensive AuNP network formation is achieved after addition of only 2 eq Hcp1_cys3 and no subsequent mixing ( Fig. 4 assembly condition C). The differences between the mean values of the length distributions (particle number) are statistically significant, but exhibit a large s.d. ( Table 1 , Supplementary Note 4 ). UV–vis spectra are in agreement with the particle size distribution ( Fig. 4a ), which can, for instance, be observed for assembly condition C. The bimodal distribution of NP-chain length shows a high abundance (29%) of smaller NP chains (10–50 NP) and 25.8% of large NP networks (10E3–100E3 NPs) and corresponds with the UV–vis spectra, depicting two local extrema at λ =534 and 637.5 nm). Thus, the extent of chain and network formation (average number of connected particles) and their associated plasmonic features can be affected by the stoichiometry and the mixing behaviour of the components. Nevertheless, the assembly conditions lead to large AuNP chain length distributions ( Fig. 4a , Supplementary Tables 3 and 4 ). Table 1 Average AuNP chain length, s.d. and P value calculated from 93 assembled structures depending on the assembly condition. Full size table Thus, by applying different assembly conditions a different anisotropic behaviour of the AuNP population is triggered. Fast mixing and excess Hcp1_cys3 addition leads to less anisotropic AuNP self-assembly. In contrast, no mixing and equimolar AuNP-Hcp1_cys3 stoichiometry induces more anisotropic AuNP assembly. Subsequently, more dipole attractions forces lead to extended AuNP coupling and a red-shifted SPR band with high intensity. AuNP chain lengths induced by three different assembly conditions can be adjusted between a few nm, several hundred nm and multiple μm ( Supplementary Fig. 6 ). Different temperatures, for example, 50 or 4 °C during the assembly process seem to have no influence (data not shown). As mentioned before, the binding characteristics of Hcp1_cys3 to individual AuNPs have been tested in depth by using the 10-nm AuNPs capped with citrate ligand only. Therefore, the maximal number of Hcp1_cys3 that are able to bind to the surface of the AuNP via its planar ring face was analysed experimentally and theoretically. Owing to the strong gold–thiol-binding energy and the dimensions of the protein corona (~4.4 nm), a planar attachment via the face of the protein ring as illustrated in Fig. 2d,f is presupposed. For complete surface coverage of the 10-nm AuNP, calculated as two-dimensional (2D) planar surface, a maximal theoretical number of 5 toroidal Hcp1_cys3-donuts was calculated ( Supplementary Note 5 ), in contrast applying the actual spherical shape of the 10-nm AuNP it was modelled, that six Hcp1_cys3 rings are required for maximal surface coverage (data not shown). To determine the surface coverage of the AuNPs experimentally, Hcp1_cys3 was titrated to an AuNP solution and the SPR was measured with UV–vis spectroscopy. Owing to protein binding to AuNPs a change of the refractive index can be monitored by a bathochromic shift of the SPR peak wavelength [40] . Using this correlation one equivalent Hcp1_cys3 ( x ) at a time was added to a solution of 10 nm AuNPs. After thoroughly mixing the maximal wavelength of the SPR peak from ( x =0 eq; 519.6±0.8 nm) up to ( x =25 eq; λ =526.2±0.5 nm) was monitored and plotted ( Fig. 5b,c ). As shown in Fig. 5b an asymptotic curvature of the regression curve towards one wavelength maximum is observed. In order to estimate the minimal number of eqs needed for complete coverage the Student’s t -test was applied. After t -test and error analysis ( Supplementary Note 6 ) one can state that ~9±3.04 equivalents of Hcp1_cys3 are needed to cover the whole surface of one AuNP of ~10 nm in diameter. This value is close to the theoretically predicted value of six molecules. The slight difference in theoretical and experimental number of molecules bound to reach saturation in surface coverage (asymptotic curvature) can be explained by multiple factors. First of all, because of thiol oxidation a greater number of Hcp1_cys3 might be needed in the titration experiment since some oxidized species do not bind immediately and accordingly do not contribute to the wavelength shift. Moreover, the protein concentration and NP concentration deviate due to variations in extinction coefficient of AuNP and Hcp1_cys3 (see Supplementary Methods ). Furthermore, the accuracy of the UV–vis spectrometer of 2 milli absorbance limits the resolution of the recorded wavelength shifts. Compared with a protein with similar size like bovine serum albumin (BSA; 5.5 × 5.5 × 9 nm) [41] it is reported that 3.7 (±0.2) × 1,012 molecules bind per cm 2.42. This implies that ~12 BSA molecules can bind to the surface of a 10-nm AuNP by an end-on mechanism. This value matches the experimentally estimated number of 9±3.04 eq Hcp1_cys3, which has comparable geometric dimensions. The knowledge about the number of attached proteins and the characterization of the Hcp1_cys3-AuNP-biohybrid system is important to build defined interaction platforms with attached functional molecules. AuNP nanoarchitecture functionalization The functionality of the NP architectures was extended via protein adaptor-encoded unnatural amino acids. Therefore, a bifunctional adapter protein, Hcp1_cys3_D11pAzF ( Fig. 1e ), was cloned and expressed. This newly designed bifunctional adapter protein allows for thiol-mediated gold conjugation and site-specific bioorthogonal conjugation of various functional molecules, for example, alkyne or cyclooctyne-modified fluorescent dyes. Hcp1cys3D11pAzF bearing the co-translational incorporated unnatural amino acid pAzF was reacted via click chemistry with two different dyes ( Fig. 6a–c ). First, the site-specific conjugation of the red chromeo alkyne dye 642 at position D11pAzF was achieved via copper-catalysed [3+2] cycloaddition between the azide and the alkyne [42] . The water-soluble Tris-[1-(3-hydroxypropyl)-1H-[1,2,3]triazol-4-yl)methyl]amine (THPTA) ligand, synthesized according to the literature [43] , protects proteins from degradation and speeds up the reaction [44] . For reaction clean up and removal of excess dye, the reaction mixture was purified by PD Spin Trap G-25 from GE Healthcare . Good coupling yields were achieved for Hcp1-Q54C-D11pAzF (80% and no precipitation) and relatively low yields for Hcp1_cys3_D11pAzF (~10–20%). The presence of numerous solvent-accessible cysteins (three thiols per subunit) leads to protein precipitation through the complexation of the thiols by copper after addition of sodium ascorbate (not observed for controls without thiols). A method, described in ref. 45 , was tried to overcome the observed site reactions. In order to prevent the copper-induced precipitation and protein degradation through formation of reactive oxygen species, excess ligand, aminoguanidine and NiCl 2 were added to the reaction. Nevertheless, the yield could not be increased. To finally overcome constraints associated with copper and sodium ascorbate [46] , a newly synthesized rhodamine dye (COMBO-rhod) [47] was attached by copper-free ring strain-promoted cycloaddition [48] between the azide-bearing unnatural amino acid and the cyclooctyne group of the dye. This reaction allows for fast site-specific conjugation without the need for copper. Successful labelling is proven via SDS–PAGE. The same gel was first excited at 250–350 nm for COMBO-rhod detection and subsequently stained with Coomassie-Brilliant Blue for protein detection ( Fig. 6d ). Labelling efficiency was calculated on the basis of the extinction coefficient of COMBO-rhod dye and protein (for details see Methods section). The labelling efficiency of freshly expressed Hcp1_cys3_D11pAzF was up to 98% but varied depending on the time gap between expression, purification and the labelling reaction. After protein storage for 6 months at 4 °C at the exclusion of light, a labelling efficiency <3% was recorded. This can be explained through azide degradation on storage. Azide-to-amine reduction is reported to be triggered in the presence of Tris[2-carboxyethyl] phosphine (TCEP) as reductant [49] , which was added to maintain the thiol of the cysteine in its reduced form. After functionalization with the dye (for example, Hcp1_cys3_D11pAzF-COMBO-rhod) the protein-adapter could successfully be attached to AuNP of various sizes. The thiol-mediated mechanism mentioned before leads to the same NP architectures functionalized with ~6 dye molecules per protein ring. This could be proven via TEM and fluorescence microscopy ( Fig. 6e,f ). The AuNP assembly into chains and networks (PABNOA) is triggered by Hcp1_cys3_D11pAzF-COMBO-rhod ( Fig. 6e ), which leads to a close proximity (~2.2 nm) of dye and AuNP. The implementation of new functional molecules (for example, dyes) into the plasmonic active NP architectures leads to strong interactions of their plasmonic features with dye vibroelectronic states. This can be detected via fluorescence microscopy and fluorescence spectroscopy by a strong quenching behaviour of ~67% after Hcp1_cys3_D11pAzF-COMBO-rhod and 10-nm AuNP incubation ( Fig. 6g ; for details see Methods section). In addition, Hcp1_cys3_D11pAzF-COMBO-rhod binding to AuNPs with 40 nm in diameter leads to less fluorescence quenching (60%). In accordance with the literature, quenching rates of fluorescent dyes critically depend on size and shape of the NP, the distance and orientation between the dye and the NP, and the overlap of the dye emission with the NP absorption band [50] . Results from other groups indicate a quenching of 50% at 10 nm (ref. 51 ) up to 99% at 1 nm (ref. 50 ) distances between AuNP and dye for AuNPs of similar size (10 and 30 nm, respectively). This is in very good agreement with our results, where 67% quenching of the dye at a distance of ~2.2 nm is observed for the 10-nm AuNP. Concordantly with ref. 52 , larger (~30 nm) AuNPs show less dye-quenching compared with smaller AuNPs (~3 nm), which is also in good agreement with the observed dye-quenching of 67% (10 nm AuNPs) and 60% (40 nm AuNPs) by us. The measured strong quenching behaviour derives from the great overlap between the emission maximum of the dye (at 586 nm) and the SPR absorption band (520 nm to ~600 nm) for the assembled 10-nm AuNPs ( Fig. 5 ). The excitation wavelength of 533 nm of the rhodamine dye does coincide with the plasmon resonance peaks of 520 and 532 nm probably leading to a decreased dye excitation because of SPR absorption. Nevertheless, this does not account for the decreased intensity of rhodamine dye photoluminescence on AuNP attachment. After attaching a fluorescein dye derivative to Hcp1_cys3_D11pAzF and binding to 10-nm AuNPs, the same quenching rate (70%) was observed even though the dye was excited at 480 nm (data not shown). Hence, decreased dye excitation due to SPR absorption plays a marginal role in the decreased photoluminescence intensity of Hcp1-dye on AuNP binding. Furthermore, once bound to the 40-nm AuNP, a strong blinking behaviour with on- and off-rates in the second scale have been observed via fluorescence microscopy ( Supplementary Movie 1 and Fig. 6f ). In contrast, no blinking is detected if COMBO-rhod dye only and 40-nm AuNPs are incubated. The group of Chriico et al . described strong blinking behaviour for a very similar dye (fluorescein derivative SAMSA) coupled to different AuNP sizes analysed with single molecule experiments [53] without protein. Such blinking effects derive from fluorophore–dipole interaction of free electrons in the metal. These interactions change the intensity and temporal and spatial distribution of the fluorophore radiation [54] . The extent of radiative versus nonradiative decay of the fluorophore emission is influenced by the fluorophore–dipole-induced electromagnetic multipole fields of the NP. A detailed discussion can be found in ref. 53 , 55 , since this goes beyond the scope of this work. Thus, control of AuNP to dye distances and assembly characteristics allow to tune subtle physical effects for biological and physical applications, which can be extended in the future. The PABNOA, introduced in this work, allows to assemble NPs with defined interparticle distance yielding different nanoarchitectures. The work described is in contrast to most existing protein-template-based NP-self-assembly schemes where NPs are organized around a given protein structure surface. We connect different NPs via a toroidal protein-donut structure selectively by genetically introducing interaction sites at defined geometric positions on the surface of the protein donut. We could demonstrate the assembly of AuNPs of different sizes into various plasmonically active biohybrid structures by means of the toroidal Hcp1 adapter protein. Assembled architectures span the range from AuNP encapsulation into the protein cavity and surface functionalization of AuNP over 1D chains and networks to ‘hedgehog’ like biohybrid nanostructures. In the current scheme using one homohexameric Hcp1 donut as NP connector, interparticle distances between NPs of 3.0 nm can be achieved. An extension to selectively conjugate two Hcp1 protein donuts yielding a toroidal protein adapter of ~8.8 nm to connect NPs with a defined inter-NP distance of ~7 nm and beyond can be envisioned. Protein-NP structures have been characterized on the molecular level by counting binding events via SPR shifts and high-resolution distance measurements via TEM. The proposed assembly mechanism involves one-sided Hcp1 to AuNP binding, which leads to dipole-driven bilateral Hcp1–AuNP assemblies. After evolving the assembly mechanism, different assembly conditions were applied to guide the extent of chain and network formation (within a large size distribution) and associated plasmonic features. Even though interparticle distance can be controlled, nanometre precise control over chain length and orientation (straight versus branched) could not be achieved yet, because of fundamental physical- and geometric effects on the nanoscale. The functionality of the different NP architectures has been extended by the design of a bifunctional (thiol and alkyne reactive) adapter protein Hcp1_cys3_D11pAzF. After successful site-selective incorporation of an unnatural amino acid, pAzF and orthogonal dye modification via click chemistry, self-assembly of the AuNP architectures via PABNOA could be induced. Blinking and quenching effects resulting from interactions of vibronic dye states and SPR of the AuNP could be observed and analysed. This emphasizes the ability to shape plasmonic/photonic and electronic interactions within complex AuNP nanostructures. These template-free grafted architectures can be used as scaffolds for the site-specific orthogonal attachment of various functional molecules, for example, enzymes for the design of enzymatic cascade reactions, biosensor applications or the assembly to functionalized surfaces. The combination of 1D nanoarchitectures and biomolecules with attached functional molecules might pave the road towards new bioelectronic devices guiding signals along 1D-assembled trajectories. Insights about the assembly mechanism and tuning of the plasmonic properties might help in the development for the fabrication of devices for subwavelength guiding, metamaterials, the transport of electromagnetic energy and bioanalytical applications. Protein expression and purification The plasmid pET 29b Hcp1_Q54C (received from the Mougous group) was transformed in E. coli BL21 (DE3) and the sequence was confirmed using sequencing (GATC sequencing facility Konstanz). E. coli strain BL21 (DE3) and E. coli stain ER2566 were used for the expression of all Hcp1 mutants. Bacteria were grown while shaking at 250 r.p.m. with 2YT medium at 37 °C until they reached OD 600 0.7. At this point, overexpression was induced with 1 μM isopropylthiogalactoside (IPTG). After 20 h at 25 °C cells were harvested with centrifugation at 4,000 g for 20 min. After suspension in lysis buffer A (500 mM NaCl, 50 mM Tris 7.5, 10% glycerol, 2 mM TCEP and 10 μg ml −1 lysozyme per litre of culture volume) the bacteria were incubated on ice for 30 min, frozen and thawn. For further purification, cells were sonified and loaded on a Ni-NTA column ( 5 PRIME ) and eluted with 150–300 mM imidazole. The concentration of Hcp1 in buffer solution was assessed using the spectrophotometer Nanodrop 1,000 from peqlab Biotechnology GmbH. The percental extinction coefficient E% of 12.98±0.65 at 280 nm obtained from ExPASy [56] was used to calculate the concentration. Spectrometry UV–vis extinction was measured with UV-VisT80+ spectrometer from pg instruments . Parameters were set to spectrum mode from 800 to 400 nm, interval=0.1 nm, speed=medium and spectral bandwidth=2 nm. Extinction of 100 μl AuNP–protein solution was recorded after blank measurement against milli Q water at 20 °C. Samples were prepared by cautious mixing of protein and 10 nM AuNP solution and incubation for at least 2 min after protein addition. Transmission electron microscopy Transmission electron microscopy (TEM) measurements were performed on a Zeiss LEO 912 Omega 120 kV. Sample volumes of 2 μl with ~10–1.83 nmo l −1 AuNP concentrations were transferred on a glow discharged carbon-coated copper grid and were allowed to dry for 5 min. For negative staining, 2 μl of 2% uranyl acetate or uranyl formate (for better resolution) was incubated for 20 s and removed with a filter paper. If not stated otherwise, sample preparation for TEM analysis involved no negative staining. Cryotransmission electron microscopy The in vitro Cryo-TEM investigations were performed with a LEO 912 OMEGA electronmicroscope (Zeiss, Oberkochen, Germany) operating at 120 kV and ‘zero-loss’ conditions. After placing a droplet (~5 μl) of the freshly prepared sample on a copper grid (Quantifoil S7/2 100 × 400 mesh, Quantifoil Micro Tools GmbH, Jena, Germany), most of the liquid was absorbed by a filter paper so that only a thin (100–500 nm) liquid film remained. The sample was then immediately shock-frozen by plunging it into liquid ethane [57] . The vitrified sample was stored at 90 K in liquid nitrogen until it was loaded into a cryogenic sample holder (D626, Gatan Inc., Pleasanton, CA). The specimens were examined at −174 °C. Digital images were recorded under low-dose conditions (MDF) with a slow-scan charge-coupled device camera system (Oxford, 1,024 × 1,024 pixel) and at minimal underfocus of the microscope objective lens to provide sufficient phase contrast [58] . Chain length size distribution The number of connected particles for each assembled structure was estimated manually for condition A and by using Image J 1.45s particle analyses tool for assembly condition B and C. For the largest assemblies (condition C), the number of connected AuNPs was estimated by calculating the 2D particle surface area, using Image J 1.45s , divided by the average 2D single-particle surface. For each condition (A—fast mixing 40 eq Hcp1_cys3; B—medium mixing 5 eq Hcp1_cys3; C—no mixing 2 eq Hcp1_cys3) 31 assembled structures ( Supplementary Table 3 ) were analysed. The frequency distribution of assembled structure length for each assembly condition was calculated by defining eight length classes (number of connected AuNPs; Supplementary Table 4 ). For statistical analysis of the AuNP chain length distributions see Supplementary Note 4 . Interparticle distance measurements High-resolution TEM images (1 pixel=0.3 nm) were recorded and the interparticle distance of 73 interacting NPs was measured. Using Image J , the plot profile and the full-width half-maximum of TEM images of assembled NP were calculated to get the maximal distances of interacting AuNP. Fluorescence microscopy Imaging of fluorescently labelled proteins Hcp1_cys3_D11pAzF-COMBO-rhod or alkyne dye 642 was carried out using epifluorescence microscopy. After expression, labelling and assembly of the desired architectures, 4 μl protein solution was transferred on a coverslip. Proteins were imaged using a NIKON eclipse TS100-F fluorescence microscope with DS-Qi1 camera and oil immersion objective CFI achromat 1.25 × 100 and the appropriate filter set-up. Images were processed using Image J 1.45s . Incorporation of pAzF Plasmids pET29Hcp1_cys3D11TAG and pEVOLpAzF (kindly provided by the Peter G. Schultz) containing the orthogonal pair of t-RNA/t-RNA synthetase (t-RNA-RS/AzPheRS for PAzF incorporation) were co-transformed into E. coli strain ER2566 NEB. For the expression of the desired protein construct Hcp1_cys3_D11pAzF, bacteria were grown while shaking at 250 r.p.m. in LB medium containing 34 μg ml −1 chloramphenicol and 40 μg ml −1 kanamycin at 37 °C until they reached an OD 600 of 0.7. At this point, 2 mM (f.c.) pAzF was added to the media. After 10-min incubation the t-RNA synthetase expression under control of an arabinose promoter was induced with 0.2% arabinose and target protein expression was triggered by adding 1 mM IPTG. After shaking for 20 h at 25 °C and 180 r.p.m., cells were harvested using centrifugation at 10,000 g for 10 min. Purification was conducted with dimed light on ice and only low concentrations of TCEP were applied to prevent an azide—amine reduction. Analysis of pAzF incorporation For LC-MS/MS analysis of the successful incorporation of PAzF into Hcp1_cys3 at D11, samples for MS analysis have been prepared by elastase in-gel digestion using a standard protocol. Extracted elastase-digested peptides were separated using nano-LC chromatography ( Dionex, Ultimate 3,000 RSLC nano system ) on C18 column ( Dionex Acclaim PepMap RSLC , 75 μm × 250 mm, C18, 2 μm, 100 Å, kept at 40 °C) at a flow rate of 300 nl min −1 . Online MS analysis was performed on ion trap Amazon Speed ETD ( Bruker Daltonics ) equipped with captive spray ion source. Voltage applied to capillary corresponded to 1.3 kV. Peptides were analysed in positive MS ion mode using enhanced resolution scan in mass range 400–3,000 m/z , with target mass focused on 900, number of precursor ions was set to 5. Singly charged ions were excluded from fragmentation. MS/MS spectra were obtained using CID fragmentation, recorded in mass range initiating at 100 m/z and finishing at m/z corresponding to the double of precursor mass. Isolation width was set to 2.2 and MS/MS fragmentation amplitude was adjusted to 60%. Spectra were annotated using Biotools 3.2 ( Bruker Daltonics ). Chemical modification of Hcp1_cys3_D11pAzF The 1,3 dipolar copper-catalysed azid-alkyne [3+2] cycloaddition also called ‘click reaction’ was carried out according to established protocols [43] . To 150 μl Hcp1_cys3_D11pAzF (f.c. 50 μmol l −1 =1 eq) in 50 mM PB pH 7.5 250 mM NaCl and 6 μl chromeo dye 642 (f.c. 333 μmol l −1 =6.5 eq). After addition of 5-μl click solution, the reaction was shaken overnight at 10 °C and 500 r.p.m. The ‘click solution’ comprises 20 eq CuSO 4 , 100 eq THPTA ligand and 200 eq Na-ascorbate. To remove excess reactants and the click solution, the reaction mixture was purified by PD Spin Trap G-25 from GE Healthcare . For the synthesis of the water-soluble THPTA ligand, see ref. 44 . Strain-promoted cycloaddition of azides and cyclooctynes . Copper-free labelling was conducted with 2–3 eq COMBO-rhod or COMBO-fluorescein at 10 °C for 2 h with 150 μl Hcp1_cys_D11pAzF (37 μM) in buffer A. To remove excess reactants, the reaction mixture was purified by PD Spin Trap G-25 from GE Healthcare. How to cite this article: Schreiber A. et al . Molecular protein adaptor with genetically encoded interaction sites guiding the hierarchical assembly of plasmonically active nanoparticle architectures. Nat. Commun. 6:6705 doi: 10.1038/ncomms7705 (2015).